CRT1 is a nuclear-translocated MORC endonuclease that participates in multiple levels of plant immunity Arabidopsis thaliana CRT1 (compromised for recognition of Turnip Crinkle Virus) was previously shown to be required for effector-triggered immunity. Sequence analyses previously revealed that CRT1 contains the ATPase and S5 domains characteristic of Microchidia (MORC) proteins; these proteins are associated with DNA modification and repair. Here we show that CRT1 and its closest homologue, CRH1, are also required for pathogen-associated molecular pattern (PAMP)-triggered immunity, basal resistance, non-host resistance and systemic acquired resistance. Consistent with its role in PAMP-triggered immunity, CRT1 interacted with the PAMP recognition receptor FLS2. Subcellular fractionation and transmission electron microscopy detected a subpopulation of CRT1 in the nucleus, whose levels increased following PAMP treatment or infection with an avirulent pathogen. These results, combined with the demonstration that CRT1 binds DNA, exhibits endonuclease activity, and affects tolerance to the DNA-damaging agent mitomycin C, argue that this prototypic eukaryotic member of the MORC superfamily has important nuclear functions during immune response activation. Plants have evolved various defenses to protect themselves from a constant barrage of potentially pathogenic microorganisms. The current model for plant disease resistance envisions a ‘zig-zag’ interplay between plant defences and pathogen counter defenses [1] . In the inoculated tissue, recognition of pathogen-associated molecular patterns (PAMPs) by extracellular surface receptors leads to activation of PAMP-triggered immunity (PTI). Although PTI is sufficient to prevent further colonization by many microbes, some pathogens have evolved effectors that suppress PTI. The resultant weak level of resistance exhibited by a host plant inoculated with such a pathogen has been defined as basal resistance [1] (it should be noted that some authors use PTI and basal resistance interchangeably [2] ). Whether such a pathogen can infect the host plant is then determined by whether the plant expresses a resistance (R) protein that directly or indirectly recognizes one of these effectors (also termed avirulence (Avr) factors) to induce effector-triggered immunity (ETI). In the absence of this Avr–R protein interaction, or if the pathogen produces additional effectors that suppress ETI, the virulence of the pathogen on its host will be promoted. Following PAMP- or R gene-mediated pathogen recognition, various defenses are activated in the infected tissue, including the accumulation of reactive oxygen species (ROS), salicylic acid (SA), and pathogenesis-related (PR) proteins [2] . ETI also is frequently associated with the development of a hypersensitive response (HR), in which necrotic lesions form at the site(s) of pathogen entry. Subsequently, PTI and ETI can trigger systemic SA accumulation and PR gene expression in the uninoculated (systemic) tissue, as well as a long-lasting, broad-based resistance to subsequent pathogen infection known as systemic acquired resistance (SAR) [2] . An additional layer of resistance, termed non-host resistance, is likely the most common form protecting plants from the thousands of microorganisms they encounter [3] . Non-host resistance appears to have a critical role in preventing non-host fungal and oomycete pathogens from penetrating host cells, as the three Arabidopsis pen ( penetration ) mutants allowed enhanced entry of Erysiphe pisi, Phytophthora infestans and/or Blumeria graminis f. sp. hordei [4] . PEN1 is a syntaxin functioning in vesicle trafficking [5] , PEN2 is a β-glucosidase [6] mainly localized in peroxisomes and PEN3 is an ATP-binding cassette transporter [4] . The mechanism involved in non-host resistance is poorly understood. However, as it often requires the signalling components EDS1, SGT1 and HSP90, as well as the hormones SA and ethylene, it appears to overlap with those for PTI and ETI [7] , [8] , [9] , [10] . Turnip Crinkle Virus (TCV) is a carmovirus that infects most Arabidopsis ecotypes. We identified a resistant ecotype, Di-17, which contains an R gene, HRT ( HR to TCV ), that triggers HR development, defence gene expression and SA accumulation following TCV infection [11] . Plants lacking HRT fail to develop an HR after TCV infection and allow systemic viral spread, followed by death of the plant [11] . A genetic screen for mutants with compromised HRT-mediated resistance identified crt1 ( compromised for recognition of TCV ) [12] . CRT1 was subsequently shown to physically interact with HRT and ten other R proteins representing three different structural classes. This interaction appears to be dynamic as CRT1 bound inactive R proteins, but only poorly interacted with activated R proteins [13] . Analysis of the Arabidopsis genome revealed that CRT1 has two close (≥70% a.a. identity) and four distant (≤50% a.a. identity) homologues. Partial silencing of CRT1’s two closest homologues, CRH1 ( CRT1 Homologue 1 ) and CRH2 , in the crt1 background compromised TCV resistance to a greater extent than that displayed by crt1 , suggesting that CRT1 and its closest homologues are functionally redundant and have an important role in ETI against TCV [12] . Cell death triggered by the R proteins ssi4 and RPS2 also was compromised by the crt1-1 mutation or silencing of CRT1 family members. Moreover, a double knockout (dKO) in the Col-0 background, crt1-2 crh1-1 , which lacks CRT1 and its closest homologue, displayed compromised resistance to avirulent Pseudomonas syringae ( Pst ) and Hyaloperonospora arabidopsidis [13] , [14] . Construction of a triple KO was not possible as the CRH2 KO was lethal in the homozygous state. Independent studies also have identified CRT1 as one of the only 11 genes whose knockout led to severe susceptibility to both virulent and avirulent H. arabidopsidis [14] . Together, these studies establish CRT1 as a key component in both ETI and basal resistance. Sequence analysis indicated that CRT1 contains a ‘GHKL’ (Gyrase, Hsp90, Histidine Kinase, MutL) ATPase motif [15] and an S5-fold domain (383aa–458aa) [16] . These domains are characteristic of MORC (Microchidia) proteins, a subset of the GHKL ATPase superfamily [16] . MORC proteins are widely distributed in eukaryotes; they also are present in a wide range of prokaryotic species, although their distribution is sporadic [16] . Mouse MORC1, the first MORC protein identified, was shown to be required for meiotic nuclear division [17] . MutL, another MORC present in prokaryotes and eukaryotes, is a key enzyme involved in initiating replacement of mismatched nucleotides on the newly synthesized DNA strand [18] . Analysis of gene neighbourhoods in prokaryoytic operons containing MORC-encoding genes further suggested that these proteins are involved in restriction modification systems, the ancient self/nonself-recognition system in prokaryotes [16] . Interestingly, two recent mutant screens for gene silencing suppressors identified Arabidopsis CRT1 and its homologue CRH6 as new factors in altering DNA/chromosome superstructure in response to epigenetic signals [19] , [20] . Here we demonstrate that CRT1 and its closest homologue, CRH1, are required for PTI, basal resistance, non-host resistance, and SAR. Immunoprecipitation (IP) assays indicated that CRT1 binds the PAMP receptor FLS2 in planta , and this interaction is not affected by flg22-induced activation of FLS2. The combined discoveries that CRT1 is a member of the MORC superfamily, a subpopulation of CRT1 is present in the nucleus, the level of nuclear-localized CRT1 increases upon activation of ETI and, to a lesser degree, PTI, CRT1 exhibits DNA/RNA-binding and endonuclease activities, and mutations in CRT1 and its closest homologue enhance tolerance to the DNA-damaging agent mitomycin C, suggest that CRT1 has an important function(s) in the nucleus, possibly associated with DNA recombination and repair (R/R) and/or chromatin structure. Together, these findings provide the first demonstration of CRT1’s function(s) at multiple levels of plant immunity, and they provide key insights into how this prototypic eukaryotic MORC functions during immune responses in plants. In turn, these results may provide important clues about the function of CRT1’s distant human counterpart in mammalian immunity. CRT1 is involved in basal resistance and PTI against viral and bacterial pathogens To assess whether CRT1 and CRH1 are required for basal resistance, TCV resistance was assessed in the dKO, which, lacks HRT . crt1-2 crh1-1 developed symptomatic chlorosis by 5 days post inoculation (d.p.i. ), whereas WT (wild type) remained green ( Fig. 1a ). Immunoblot (IB) analysis indicated that crt1-2 crh1-1 supported substantially greater TCV replication than WT, as the dKO contained 12.7-fold more coat protein (CP) in the inoculated leaves than WT at 3 d.p.i. ( Fig. 1b ). Fourteen-fold more CP was also detected in the uninoculated tissue of the dKO compared with that in WT, indicating that the virus spread and replicated more readily in the dKO. In addition, the dKO supported 2.7-fold more growth of virulent Pst than WT plants ( Fig. 1c , compare mock-pretreated WT versus crt1-2 crh1-1 ). 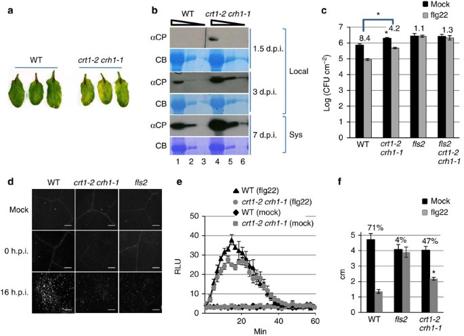Figure 1: Basal resistance and PTI against TCV andP. syringaeis compromised incrt1-2 crh1-1. (a) TCV-inoculated leaves were excised from 4-week-old WT andcrt1-2 crh1-1plants and photographed at 5 d.p.i. (b) Quantification of TCV CP using IB analysis with αCP antibody was performed with two 10-fold serial dilutions from 1 to 100 of the protein extracts. Protein extracts were prepared from inoculated leaves (Local) at 1.5 and 3 d.p.i. with TCV, and from systemic leaves (Sys) at 7 d.p.i.. Coomassie blue staining (CB) was performed as a loading control. This experiment was done three times with similar results. (c) Four-week-old plants from the indicated lines were pretreated with water (mock) or 0.2 μM flg22 for 1 day and inoculated withPst(105c.f.u. ml−1). Bacterial growth was determined 3 d.p.i.. The mean±s.e. values are presented (n=4). The fold reduction (mock/flg22) is indicated at the top of the bars. Asterisks indicate statistical difference from WT or in the fold reduction between WT andcrt1-2 crh1-1; *P<0.05 (t-tests). Similar results were observed in three independent experiments. (d) Callose deposition was visualized in WT,crt1-2 crh1-1andfls2plants by aniline blue staining at 0 and 16 h.p.i. withPst hrcC(105c.f.u. ml−1). Mock control plants were stained 16 h post syringe infiltration with MgCl2. Scale bar, 100 μm. This experiment was done twice with similar results. (e) Oxidative burst induced by water (mock), or 1 μM flg22 treatment was measured in relative light units (RLU) in the leaves of WT andcrt1-2 crh1-1at the times indicated. The mean±s.e. values are presented (n=6). An independent experiment was performed with a similar result. (f) Root length of the indicated lines germinated and grown for 10 days in liquid Murashige Skoog (MS) medium containing 0 (mock) or 1 μM flg22. The mean±s.e. values are presented (n=6). Statistical difference from WT is indicated; *P<0.05 (t-test). The reduction in percentage (flg22/mock) is indicated at the top of the bars. This experiment was done twice with similar results. Figure 1: Basal resistance and PTI against TCV and P. syringae is compromised in crt1-2 crh1-1 . ( a ) TCV-inoculated leaves were excised from 4-week-old WT and crt1-2 crh1-1 plants and photographed at 5 d.p.i. ( b ) Quantification of TCV CP using IB analysis with αCP antibody was performed with two 10-fold serial dilutions from 1 to 100 of the protein extracts. Protein extracts were prepared from inoculated leaves (Local) at 1.5 and 3 d.p.i. with TCV, and from systemic leaves (Sys) at 7 d.p.i.. Coomassie blue staining (CB) was performed as a loading control. This experiment was done three times with similar results. ( c ) Four-week-old plants from the indicated lines were pretreated with water (mock) or 0.2 μM flg22 for 1 day and inoculated with Pst (10 5 c.f.u. ml −1 ). Bacterial growth was determined 3 d.p.i.. The mean±s.e. values are presented ( n =4). The fold reduction (mock/flg22) is indicated at the top of the bars. Asterisks indicate statistical difference from WT or in the fold reduction between WT and crt1-2 crh1-1 ; * P <0.05 ( t -tests). Similar results were observed in three independent experiments. ( d ) Callose deposition was visualized in WT, crt1-2 crh1-1 and fls2 plants by aniline blue staining at 0 and 16 h.p.i. with Pst hrcC (10 5 c.f.u. ml −1 ). Mock control plants were stained 16 h post syringe infiltration with MgCl 2 . Scale bar, 100 μm. This experiment was done twice with similar results. ( e ) Oxidative burst induced by water (mock), or 1 μM flg22 treatment was measured in relative light units (RLU) in the leaves of WT and crt1-2 crh1-1 at the times indicated. The mean±s.e. values are presented ( n =6). An independent experiment was performed with a similar result. ( f ) Root length of the indicated lines germinated and grown for 10 days in liquid Murashige Skoog (MS) medium containing 0 (mock) or 1 μM flg22. The mean±s.e. values are presented ( n =6). Statistical difference from WT is indicated; * P <0.05 ( t -test). The reduction in percentage (flg22/mock) is indicated at the top of the bars. This experiment was done twice with similar results. Full size image Flagellin is a PAMP that is present in a broad range of bacterial pathogens, including Pst [21] ; it triggers the induction of numerous defence-related genes and resistance to pathogens [22] . To assess whether flagellin-induced PTI requires CRT1, WT and dKO plants were pretreated with an epitope of flagellin, flg22, and then infected with Pst . Reduction in Pst growth due to flg22 pretreatment was 50% less in the dKO than in WT ( Fig. 1c ), indicating that flg22-induced PTI was partially compromised. Please note that the modest reduction in basal resistance/PTI exhibited by crt1-2 crh1-1 is likely due to the presence of CRH2, which complements the original crt1-1 mutant (unpublished, H.G.K. and D.F.K.). FLS2 is the receptor that recognizes flagellin [23] . To assess the genetic interaction between FLS2 and CRT1 in PTI, a fls2-101 crt1-2 crh1-1 triple mutant was generated and challenged with Pst . As expected, the fls2 single mutant displayed increased susceptibility to Pst [22] , and pretreatment with flg22 induced little resistance ( Fig. 1c ). Similar levels of bacterial growth were observed in mock- and flg22-pretreated triple mutant plants, suggesting that CRT1 and FLS2 function in the same defence signalling pathway. Whether CRT1 and CRH1 are required for other FLS2-mediated responses was then assessed. Callose deposition, a hallmark of FLS2-mediated PTI, was monitored by inoculating plants with non-pathogenic Pst hrcC , which lacks a functional type III secretion apparatus (an effector delivery system) but carries a collection of PAMPs sufficient to trigger callose deposition [24] . In comparison with WT plants, callose deposition after Pst hrcC infection was reduced about 80% in the dKO and fls2 mutants ( Fig. 1d ; Supplementary Fig. S1a ). As enhanced ROS generation is one of the earliest events induced after FLS2 activation by flg22, ROS levels were monitored after flg22 or mock treatment. The dKO displayed reduced ROS generation compared with WT ( Fig. 1e ; Supplementary Fig. S1b ); the total ROS accumulation for 30 min after 1 μM flg22 treatment was 19% lower in the dKO as compared with that in WT ( Supplementary Fig. S1c ). Continuous activation of FLS2-mediated defence responses due to the presence of flg22 was previously shown to retard root growth in WT, but not fls2 plants [23] . Analysis of the dKO revealed that flg22-induced root growth retardation also was compromised ( Fig. 1f ; Supplementary Fig. S1d ). Together, these results indicate that the CRT1 family affects a broad range of PTI responses. However, the reduced PTI exhibited by dKO plants does not appear to be caused by significant alterations in the transcriptome. Using quantitative real-time RT–PCR, the expression of four widely used PTI marker genes ( MYB51 , PAD3 , PAL1 and FRK) [25] and seven CRA ( CRT1-associated ) genes (which are differentially expressed in dKO versus WT plants in response to avirulent Pst AvrRpt2 (ref. 13 )) was monitored in mock- and flg22-treated dKO and WT plants. Only PAD3 and CRA2 showed small, but statistically significant, reductions in flg22-induced expression in the dKO compared with WT ( Supplementary Fig. S2 ). CRT1 is involved in non-host resistance and SAR To investigate whether CRT1 and CRH1 are required for non-host resistance, we monitored symptom severity, the levels of cell death, callose deposition and penetration attempts in dKO and WT plants after P. infestans inoculation. The dKO exhibited elevated levels of chlorosis and cell death, almost comparable to the heightened levels observed in pen2-2 (ref. 7 ), whereas little to no cell death was detected in WT ( Fig. 2a ). Callose deposition, which is activated in non-host pathogen-inoculated WT, but not in pen2-2 (ref. 6 ), also was compromised in the dKO ( Fig. 2c ; Supplementary Fig. S3 ). Another measure of non-host resistance is the frequency of successful penetration attempts with initiation of haustoria formation. In contrast to WT, where 75% or more of the leaves had few, if any, detectable penetration attempts, more than half of the dKO or pen2-2 leaves had high numbers of successful attempts resulting in haustorium initials ( Fig. 2d ). Together, these results argue that the CRT1 family also has a role in non-host resistance. 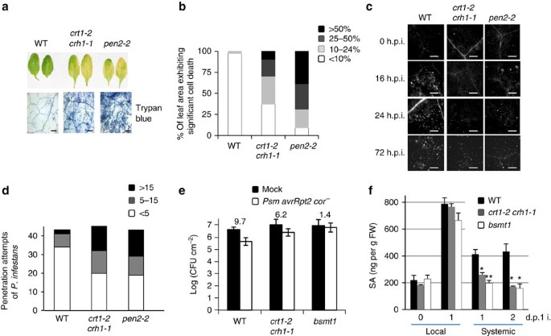Figure 2:crt1-2 crh1-1is compromised for non-host resistance toP. infestansand SAR toP. syringae. (a) Four-week-old WT,crt1-2 crh1-1andpen2-2plants were spray-inoculated with a sporangia suspension (1 × 105sporangia per ml) ofP. infestans. Leaves were photographed 3 d.p.i. (top panel) and stained with trypan blue to visualize cell death (lower panel). Scale bar, 0.5 mm. (b) Quantification of cell death in the indicated lines at 3 d.p.i. withP. infestans. The percentage of leaf area exhibiting cell death was determined using a total of 27 leaves from nine plants per genotype. (c) Callose deposition was visualized in the indicated lines by staining pathogen-inoculated leaves with aniline blue at 0, 16, 24 or 72 h.p.i.. Scale bar, 100 μm. (d) Total number ofP. infestanspenetration attempts in each of the indicated lines was determined using ~50 inoculated leaves collected 16, 24 and 72 h.p.i. incafter staining with aniline blue. (e) SAR was monitored in WT,crt1-2 crh1-1orbsmt1plants by performing a primary infection with MgCl2(mock) or avirulentPsm AvrRpt2 cor−, and subsequently inoculating two systemic, uninoculated leaves with virulentPst.The growth of virulentPstwas determined at 3 days post secondary infection. The mean±s.e. values are presented (n≥5). The fold reduction (mock/Psm-avrRpt2 cor−) is indicated at the top of the bars. Two independent experiments were analysed with similar results. (f) SA content was quantified in the inoculated leaves of 3–4-week-old plants at 0 and 1 day post primary infection (d.p.1 i.) withPsm AvrRpt2cor−and in the uninoculated leaves at 1 and 2 d.p.1 i. The mean±s.e. values are presented (n=40). Experiments were done twice with the similar results. Asterisks indicate statistically significant differences (**P<0.01, *P<0.05,t-test) between mutants and WT. Figure 2: crt1-2 crh1-1 is compromised for non-host resistance to P. infestans and SAR to P. syringae . ( a ) Four-week-old WT, crt1-2 crh1-1 and pen2-2 plants were spray-inoculated with a sporangia suspension (1 × 10 5 sporangia per ml) of P. infestans . Leaves were photographed 3 d.p.i. (top panel) and stained with trypan blue to visualize cell death (lower panel). Scale bar, 0.5 mm. ( b ) Quantification of cell death in the indicated lines at 3 d.p.i. with P. infestans . The percentage of leaf area exhibiting cell death was determined using a total of 27 leaves from nine plants per genotype. ( c ) Callose deposition was visualized in the indicated lines by staining pathogen-inoculated leaves with aniline blue at 0, 16, 24 or 72 h.p.i.. Scale bar, 100 μm. ( d ) Total number of P. infestans penetration attempts in each of the indicated lines was determined using ~50 inoculated leaves collected 16, 24 and 72 h.p.i. in c after staining with aniline blue. ( e ) SAR was monitored in WT, crt1-2 crh1-1 or bsmt1 plants by performing a primary infection with MgCl 2 (mock) or avirulent Psm AvrRpt2 cor − , and subsequently inoculating two systemic, uninoculated leaves with virulent Pst. The growth of virulent Pst was determined at 3 days post secondary infection. The mean±s.e. values are presented ( n ≥5). The fold reduction (mock/ Psm-avrRpt2 cor − ) is indicated at the top of the bars. Two independent experiments were analysed with similar results. ( f ) SA content was quantified in the inoculated leaves of 3–4-week-old plants at 0 and 1 day post primary infection (d.p.1 i.) with Psm AvrRpt2 cor − and in the uninoculated leaves at 1 and 2 d.p.1 i. The mean±s.e. values are presented ( n =40). Experiments were done twice with the similar results. Asterisks indicate statistically significant differences (** P <0.01, * P <0.05, t -test) between mutants and WT. Full size image Whether CRT1/CRH1 also function in SAR was investigated by inoculating three lower leaves of WT, dKO or SAR-deficient bsmt1 ( benzoic acid/SA methyl transferase ) [2] plants with either buffer (mock) or P. syringae pv. maculicola ( Psm ) AvrRpt2 cor − . Resistance to a subsequent inoculation with virulent Pst was then monitored. Growth of virulent Pst was reduced 9.7-fold in SAR-induced WT, which had received a primary inoculation with Psm AvrRpt2 cor − , as compared with the mock-inoculated control ( Fig. 2e ), whereas little reduction in Pst growth was observed in bsmt1 . Pst growth in dKO that received a primary infection with Psm AvrRpt2 cor − was 6.2-fold lower than that in mock-inoculated dKO, indicating that SAR is partially compromised. Pathogen infection induces SA accumulation in the local and systemic leaves; the increase in uninoculated leaves correlates strongly with SAR development [2] . CRT1/CRH1 do not appear to be required for local SA accumulation in response to Pst avrRpt2 cor − , as SA levels in the inoculated leaves of dKO and WT plants were comparable at 1 d.p.1 i. ( Fig. 2f ). However, SA was significantly reduced in the systemic leaves of both dKO and bsmt1 as compared with WT (2.5-and 2.7-fold in dKO and bsmt at 2 d.p.1 i., respectively). Together, these results indicate that the CRT1 family is required for full SAR development. CRT1 physically associates with FLS2 in planta To assess whether CRT1 and FLS2 interact, these proteins were tagged with Myc and Flag epitopes, respectively, and then co-expressed in Nicotiana benthamiana via Agro-infiltration. IP of FLS2-Flag using αFlag antibodies revealed that CRT1 physically associates with FLS2, whereas the negative control, Myc-GFP, did not ( Fig. 3a ). Reciprocal IP of Myc-CRT1 using αMyc antibodies confirmed that FLS2 physically associates with CRT1 ( Supplementary Fig. S4 ). Interestingly, although activation of R proteins was previously shown to disrupt the R protein–CRT1 interaction [21] , CRT1 remained physically associated with FLS2 after flg22 treatment ( Fig. 3a ). Thus, the CRT1–FLS2 interaction may be less dynamic. 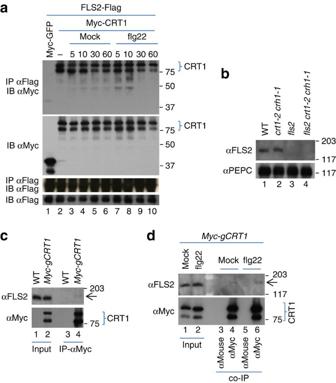Figure 3: CRT1 physically associates with FLS2. (a)Myc-CRT1,Myc-GFPandFLS2-Flagwere transiently overexpressed for 2 days inN. benthamiana. After water (mock) or flg22 (1 μM) treatment for the indicated times (min), protein extracts were prepared and either subjected to (i) 12% SDS–PAGE followed by IB analysis with the indicated antibodies, or (ii) co-IP with αFlag antibody conjugated to beads, followed by IB analysis with αMyc antibodies. A bracket indicates the expected size of the CRT1 doublet. (−) denotes the untreated control. Independent experiments were performed twice with similar results. (b) IB analysis with αFLS2 antibody was performed with protein extracts prepared from the indicatedArabidopsislines. αPEPC was used to assess sample loading. (c) IB analysis using αFLS2 or αMyc antibodies was performed with protein extracts (input) prepared from WT orMyc-gCRT1plants or following co-IP with agarose-conjugated αMyc antibody from these proteins extracts. (d)Myc-gCRT1plants were treated with water (mock) or flg22 (1 μM) for 30 min. Protein extracts were prepared and then subjected to IB analysis with αFLS2 and αMyc antibodies before (input) or after co-IP with agarose-conjugated αMyc or αMouse antibodies. An arrow indicates the expected size of FLS2 (c,d). (a–d) Size markers are shown at the right of the panels in kDa. Figure 3: CRT1 physically associates with FLS2. ( a ) Myc-CRT1 , Myc-GFP and FLS2-Flag were transiently overexpressed for 2 days in N. benthamiana . After water (mock) or flg22 (1 μM) treatment for the indicated times (min), protein extracts were prepared and either subjected to (i) 12% SDS–PAGE followed by IB analysis with the indicated antibodies, or (ii) co-IP with αFlag antibody conjugated to beads, followed by IB analysis with αMyc antibodies. A bracket indicates the expected size of the CRT1 doublet. (−) denotes the untreated control. Independent experiments were performed twice with similar results. ( b ) IB analysis with αFLS2 antibody was performed with protein extracts prepared from the indicated Arabidopsis lines. αPEPC was used to assess sample loading. ( c ) IB analysis using αFLS2 or αMyc antibodies was performed with protein extracts (input) prepared from WT or Myc-gCRT1 plants or following co-IP with agarose-conjugated αMyc antibody from these proteins extracts. ( d ) Myc-gCRT1 plants were treated with water (mock) or flg22 (1 μM) for 30 min. Protein extracts were prepared and then subjected to IB analysis with αFLS2 and αMyc antibodies before (input) or after co-IP with agarose-conjugated αMyc or αMouse antibodies. An arrow indicates the expected size of FLS2 ( c , d ). ( a – d ) Size markers are shown at the right of the panels in kDa. Full size image The co-chaperones HSP90 and SGT1 are important for R protein stability, as well as for ETI [26] , [27] ; thus, the compromised resistance in hsp90 and sgt1 is likely due to R protein instability [26] . In comparison, CRT1 does not seem to affect the stability of R proteins; RPS2 levels in the dKO were comparable to those in WT [13] . Consistent with this finding, IB analysis revealed comparable levels of FLS2 in WT and dKO ( Fig. 3b ). No FLS2 was detected in the fls2 or triple mutant, confirming the specificity of the αFLS2 antibody. Owing to the difficulty in detecting immune receptors at their low endogenous levels, CRT1’s interaction with immunity receptors was previously demonstrated using proteins transiently overexpressed in N. benthamiana . However, as the αFLS2 antibody detected endogenous FLS2, the interaction between FLS2 and Myc-tagged genomic CRT1, which was expressed at physiological levels under its own promoter in the dKO background ( Myc-gCRT1 ), was monitored. Note that CRT1 tagged with Myc at its N terminus is fully functional, as it complemented the crt1-1 phenotype [12] . A small quantity of FLS2 was found to co-IP with Myc-CRT1 ( Fig. 3c ). Note that FLS2 co-IP with CRT1 migrated ~5 kDa slower than input-FLS2 (for example compare lanes 2 versus 4 in Fig. 3c ), suggesting that FLS2 interacting with CRT1 is post-translationally modified. To establish the specificity of this CRT1–FLS2 interaction, agarose-conjugated αMouse antibody was used in the co-IP assay with protein extracts prepared from Myc-gCRT1. In comparison with αMyc, the αMouse antibody failed to co-IP FLS2 ( Fig. 3d , lanes 3 and 5 versus 4 and 6). Consistent with the results in Fig. 3a , pretreatment with flg22 did not reduce the CRT1–FLS2 interaction ( Fig. 3d ). Together, these results indicate that CRT1 physically associates with FLS2 expressed at physiological levels, and that this interaction is not disrupted by FLS2 activation. Activation of immune receptors enhances CRT1 accumulation in the nucleus As CRT1 family members contain two domains characteristic of MORCs, and eukaryotic MORC proteins are associated with the nucleus, the presence of CRT1 in the nucleus was examined. Using Myc-gCRT1 leaves, transmission electron microscopy (TEM) via indirect immunogold labelling revealed immune reactivity with αMyc in cytosolic microbodies/endomembrane-like vesicles ( Supplementary Fig. S5a ), consistent with earlier immunofluorescence analyses using GFP-tagged CRT1(ref. 13 ). TEM also detected CRT1, represented by the gold labels, in the nuclei of mock- and flg22-treated leaves ( Fig. 4a–f ). In mock-treated leaves, the nuclear-localized gold labels were evenly distributed, mainly as single particles associated with filamentous, grey structures representing euchromatin fibres. Clustering of gold labels was rarely visible and did not exceed four particles per cluster ( Fig. 4b and Supplementary Fig. S6d ). A comparable labelling pattern was observed in nuclei from untreated Myc-gCRT1 transgenic plants ( Supplementary Fig. S5b ). Following flg22 treatment, the number of nuclear-localized gold labels, and the number of clusters containing three or more particles, increased significantly ( Fig. 4c–g ; Supplementary Fig. S6a–d ). In addition, single particles and clusters of gold label were observed near the nuclear pores of flg22-treated plants, perhaps reflecting nuclear-cytosol shuttling of CRT1 ( Supplementary Fig. S7 ); please note that the postulated shuttle may be rapid, as immunolabelling of nuclear pores was a rare event, which could not be validated by statistical analysis. 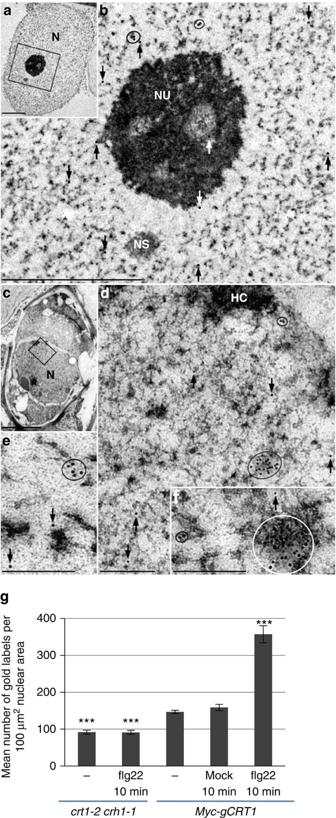Figure 4: TEM detects CRT1 in the nucleus. Indirect immunogold labelling was performed on leaf tissues of 6-week-oldMyc-gCRT1using αMyc Mouse antibodies to detect Myc-tagged CRT1, followed by αMouse antibodies conjugated to gold particles. Single gold labels are denoted with arrows, and circles mark clusters of more than one gold label. (a) Nucleus (N) of a mesophyll cell 10 min post treatment with 10 mM MgCl2(mock). (b). Higher magnification of the nuclear region and nucleolus (NU) contained in the boxed area shown ina. The diameter of the 5 nm gold labels were enlarged two-fold to enhance visibility. NS, putative nuclear speckle of relatively large size. (c) N in a phloem parenchyma cell 10 min post infiltration with 5 μM flg22. (d) Higher magnification of the nuclear region contained in the boxed area shown inc. HC, heterochromatin. (e,f) Regions of mesophyll cell and phloem parenchyma nuclei 10 min post infiltration with 5 μM flg22 containing large clusters of CRT1. Scale bars, 2 μm (a–c), 200 nm (d–f). (g) Mean number of gold labels per 100 μm2nucleus area ofMyc-gCRT1after treatment with 10 mM MgCl2(mock) or 5 μM flg22 for the indicated times. (−) denotes no treatment.crt1-2 crh1-1, which lacks theMyc-gCRT1transgene, served as a negative control. The mean±s.e. values are presented (n≥33). Asterisks indicate statistically significant difference (***P<0.001, Mann–Whitney test) to theMyc-gCRT1mock control. Figure 4: TEM detects CRT1 in the nucleus. Indirect immunogold labelling was performed on leaf tissues of 6-week-old Myc-gCRT1 using αMyc Mouse antibodies to detect Myc-tagged CRT1, followed by αMouse antibodies conjugated to gold particles. Single gold labels are denoted with arrows, and circles mark clusters of more than one gold label. ( a ) Nucleus (N) of a mesophyll cell 10 min post treatment with 10 mM MgCl 2 (mock). ( b ). Higher magnification of the nuclear region and nucleolus (NU) contained in the boxed area shown in a . The diameter of the 5 nm gold labels were enlarged two-fold to enhance visibility. NS, putative nuclear speckle of relatively large size. ( c ) N in a phloem parenchyma cell 10 min post infiltration with 5 μM flg22. ( d ) Higher magnification of the nuclear region contained in the boxed area shown in c . HC, heterochromatin. ( e , f ) Regions of mesophyll cell and phloem parenchyma nuclei 10 min post infiltration with 5 μM flg22 containing large clusters of CRT1. Scale bars, 2 μm ( a – c ), 200 nm ( d – f ). ( g ) Mean number of gold labels per 100 μm 2 nucleus area of Myc-gCRT1 after treatment with 10 mM MgCl 2 (mock) or 5 μM flg22 for the indicated times. (−) denotes no treatment. crt1-2 crh1-1 , which lacks the Myc-gCRT1 transgene, served as a negative control. The mean±s.e. values are presented ( n ≥33). Asterisks indicate statistically significant difference (*** P <0.001, Mann–Whitney test) to the Myc-gCRT1 mock control. Full size image The presence of a CRT1 subpopulation in the nucleus was confirmed using subcellular fractionation. In mock-treated Myc - gCRT1 plants, the nucleus-enriched subcellular fractions contained very low levels of CRT1; ~2-fold greater levels were detected in the nucleus-enriched fractions from flg22-treated plants ( Fig. 5a ). Similarly, nuclear CRT1 levels were ~2-fold higher in Pst hrcC- inoculated Myc - gCRT1 plants than in mock-inoculated plants at 30 min after infection ( Supplementary Fig. S8 ). As FLS2 activation appears to lead to rapid, modest increases in nuclear CRT1, we tested whether other types of immune activation also influence nuclear CRT1 levels. Interestingly, subcellular fractionation revealed ~9-fold increase in nuclear CRT1 by 16 h post inoculation (h.p.i.) with avirulent Pst AvrRpt2 ( Fig. 5b ); this time point was chosen to ensure that ETI was fully activated. By contrast, no increase in nuclear CRT1 levels was detected at 16 h.p.i. with virulent Pst or Pst hrcC . These results indicate that ETI, which triggers the strongest immune response, also promotes the greatest translocation of CRT1 to the nucleus, whereas PTI induces a modest, rapid, and transient increase in nuclear CRT1. 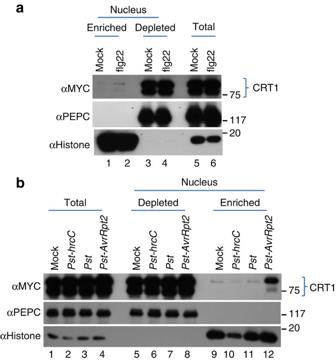Figure 5: Nuclear localization of CRT1 is enhanced by a PAMP treatment or activation of ETI. (a) Subcellular fractionation was performed onMyc-gCRT1plants that received water (mock) or 1 μM flg22 treatment for 30 min. IB analysis with αMyc antibodies was carried out with total, nucleus-depleted and nucleus-enriched (20 × ) fractions. Antibodies against histone H3 and PEPC (phosphoenolpyruvate carboxylase), a nuclear and a cytosolic protein, respectively, were used to ensure appropriate enrichment or depletion of nuclei. (b) Subcellular fractionation was performed onMyc-gCRT1treated with mock,Pst hrcC, PstorPst AvrRpt2(106c.f.u. ml−1) at 16 h.p.i. IB analysis was carried out as described ina. (a,b) Size markers are shown at the right of the panels in kDa. Figure 5: Nuclear localization of CRT1 is enhanced by a PAMP treatment or activation of ETI. ( a ) Subcellular fractionation was performed on Myc-gCRT1 plants that received water (mock) or 1 μM flg22 treatment for 30 min. IB analysis with αMyc antibodies was carried out with total, nucleus-depleted and nucleus-enriched (20 × ) fractions. Antibodies against histone H3 and PEPC (phosphoenolpyruvate carboxylase), a nuclear and a cytosolic protein, respectively, were used to ensure appropriate enrichment or depletion of nuclei. ( b ) Subcellular fractionation was performed on Myc-gCRT1 treated with mock, Pst hrcC, Pst or Pst AvrRpt2 (10 6 c.f.u. ml −1 ) at 16 h.p.i. IB analysis was carried out as described in a . ( a , b ) Size markers are shown at the right of the panels in kDa. Full size image CRT1 is a DNA-binding protein with endonuclease activity As most eukaryotic and prokaryotic MORC proteins are associated with nucleic acid-modifying activities, we tested whether CRT1 binds DNA and RNA. Nucleic acid binding, when mediated by Trp-residues, can cause a change in the intrinsic fluorescence [28] ; thus, the fluorescence of CRT1 in the absence/presence of two different DNAs and RNAs was monitored. TCV DNA and RNA were included in the binding assay to assess whether CRT1 specifically interacts with them, as TCV resistance requires CRT1. All four nucleic acids quenched the intrinsic fluorescence of recombinant CRT1 ( Fig. 6a ), suggesting that CRT1 likely interacts with DNA/RNA in a nonspecific manner. This quenching was greatly suppressed when CRT1 was denatured ( Fig. 6b ). 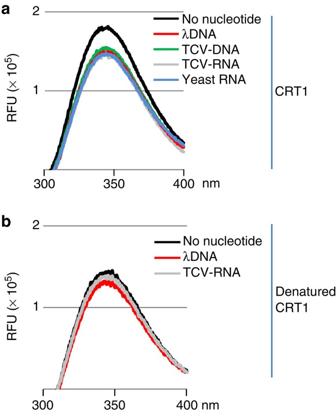Figure 6: CRT1 is a DNA-binding protein. Trp-fluorescence in relative fluorescence unit (RFU) of recombinant CRT1 protein in the native (a) or denatured (b) state was monitored in the presence/absence of 100 ng of the indicated nucleic acid. Figure 6: CRT1 is a DNA-binding protein. Trp-fluorescence in relative fluorescence unit (RFU) of recombinant CRT1 protein in the native ( a ) or denatured ( b ) state was monitored in the presence/absence of 100 ng of the indicated nucleic acid. Full size image Whether CRT1 exhibits endonuclease activity was then investigated by monitoring the conformation/integrity of supercoiled plasmid DNA after incubation with highly purified recombinant CRT1. To help insure that the endonuclease activity being observed was due to CRT1 rather than a contaminating endonuclease, a couple of precautions were taken. First, recombinant His-tagged CRT1 was subjected to three purification steps including nickel-based affinity chromatography, size fractionation by gel filtration chromatography, and anion exchange chromatography. Second, as a negative control, a truncated version of CRT1 (CRT1-CC) carrying the predicted coil-coiled domain (511–635 a.a.) was purified in parallel with full-length CRT1 and tested for endonuclease activity. Note that coil-coiled domains are often involved in protein–protein interactions, nonspecific as well as specific. In the presence of increasing concentrations of CRT1 or increasing incubation times, the level of supercoiled plasmid DNA was correspondingly reduced ( Fig. 7 ). Analysis of endonuclease activity in the presence of different divalent cations revealed that CRT1 exhibits a strong preference for Mn 2+ and, to a lesser degree, Mg 2+ as a metal cofactor ( Fig. 7a ). In contrast, little if any endonuclease activity was associated with truncated CRT1-CC ( Fig. 7 ). Together, these results argue that CRT1 is a nucleic acid-interacting protein with endonuclease activity. 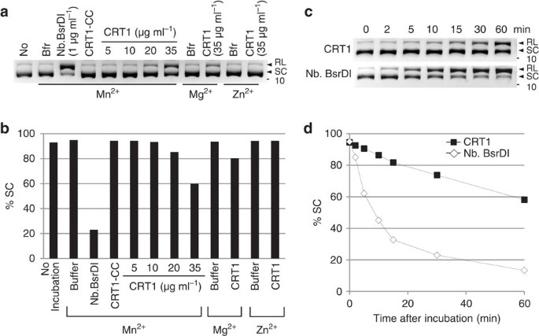Figure 7: CRT1 displays a Mn2+-dependent endonuclease activity. (a) Endonuclease activities of purified recombinant CRT1, its truncated mutant CRT1-CC and Nb.BsrDI, a positive control, were determined in the presence of 10 mM MnCl2, MgCl2or ZnCl2. Following incubation with plasmid DNA, supercoiled (SC) and relaxed (RL) DNA was resolved on a 1.2% agarose gel. The no incubation (No) and buffer only (Bfr) lanes contain plasmid DNA that was electrophoresed either immediately after CRT1 protein addition or in the absence of CRT1 protein, respectively. Note that the amount of CRT1-CC used inawas equivalent to 140 μg ml−1CRT1 on a per molar basis. (b) Percentage of SC plasmid DNA remaining after the reactions shown ina. (c) Time-dependent degradation of plasmid DNA by CRT1 (35 μg ml−1) or Nb.BsrDI (1 μg ml−1) in the presence of 10 mM MnCl2. (d) Percentage of SC plasmid DNA remaining at different times during the reaction shown inc. Two independent experiments were performed with similar results. (a,c) Size markers are shown at the right of the panels in kb. Figure 7: CRT1 displays a Mn 2+ -dependent endonuclease activity. ( a ) Endonuclease activities of purified recombinant CRT1, its truncated mutant CRT1-CC and Nb.BsrDI, a positive control, were determined in the presence of 10 mM MnCl 2 , MgCl 2 or ZnCl 2 . Following incubation with plasmid DNA, supercoiled (SC) and relaxed (RL) DNA was resolved on a 1.2% agarose gel. The no incubation (No) and buffer only (Bfr) lanes contain plasmid DNA that was electrophoresed either immediately after CRT1 protein addition or in the absence of CRT1 protein, respectively. Note that the amount of CRT1-CC used in a was equivalent to 140 μg ml −1 CRT1 on a per molar basis. ( b ) Percentage of SC plasmid DNA remaining after the reactions shown in a . ( c ) Time-dependent degradation of plasmid DNA by CRT1 (35 μg ml −1 ) or Nb.BsrDI (1 μg ml −1 ) in the presence of 10 mM MnCl 2 . ( d ) Percentage of SC plasmid DNA remaining at different times during the reaction shown in c . Two independent experiments were performed with similar results. ( a , c ) Size markers are shown at the right of the panels in kb. Full size image The CRT1 family affects tolerance to mitomycin C Endonucleases, including the MORC protein MutL, have critical roles in DNA R/R [16] , [18] , [29] . To assess whether CRT1/CRH1 are involved in DNA R/R, the dKO was monitored for altered resistance to the DNA-damaging agent, mitomycin C. Consistent with earlier studies, WT plants grown in the presence of mitomycin C exhibited reduced ability to form true leaves [30] . True leaf formation in dKO plants was suppressed to a lesser extent than in WT ( Fig. 8 ; 43% of WT versus 72% of dKO at 80 mM mitomycin C), indicating enhanced mitomycin C tolerance. By contrast, the suppressor of sni1 1 ( ssn1 ) mutant, which carries a mutation in RAD51, a key factor in R/R, was hypersensitive to mitomycin C, as previously reported [30] . This result indicate that the CRT1 family is involved in DNA repair, perhaps as a negative regulator. 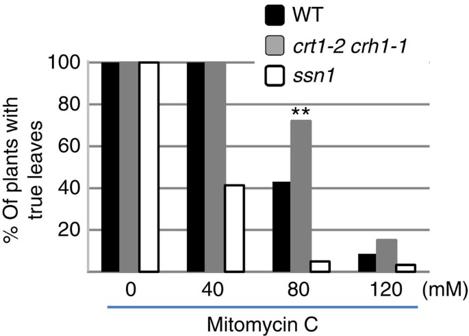Figure 8:crt1-2 crh1-1displays enhanced tolerance to a DNA-damaging agent. Tolerance to the DNA-damaging agent mitomycin C was assessed in WT,crt1-2 crh1-1andssn1plants by monitoring true leaf development in the presence of increasing concentrations of mitomycin C. The statistical difference from WT is indicated;**P<0.01 (Fisher’s exact test). Minimum 30 plants/genotypes were used for each treatment. Two independent experiments gave similar results. Figure 8: crt1-2 crh1-1 displays enhanced tolerance to a DNA-damaging agent. Tolerance to the DNA-damaging agent mitomycin C was assessed in WT, crt1-2 crh1-1 and ssn1 plants by monitoring true leaf development in the presence of increasing concentrations of mitomycin C. The statistical difference from WT is indicated; ** P <0.01 (Fisher’s exact test). Minimum 30 plants/genotypes were used for each treatment. Two independent experiments gave similar results. Full size image In this study, we extend our previous findings to show that CRT1 is involved in multiple levels of the immune response. In addition, TEM and subcellular fractionation revealed that a subpopulation of CRT1 is present in the nucleus, and that nuclear CRT1 levels increase following activation of PTI or ETI. Consistent with its nuclear location, CRT1 exhibited DNA-binding and Mn 2+ -dependent endonuclease activities, which are also found in the MORC protein MutL [29] . These findings, together with CRT1’s membership in the MORC superfamily, suggest that it has a role in modifying chromatin/DNA, as shown for animal MORC proteins, including MutL and MORC1 (refs 18 , 31 ). CRT1 interacts in planta with a large number of proteins involved in plant immunity when they are co-expressed in N. benthamiana [12] , [13] ( Fig. 3 ). Recent Arabidopsis genome-wide interactome studies have confirmed these interactions, and suggest that they are indirect, mediated via two bridging proteins [32] , [33] . Consistent with these results, a yeast two-hybrid system did not detect direct interaction between CRT1 and R proteins or PAMP-recognition receptors (PRRs; unpublished, H.G.K. and D.F.K.). As FLS2 is predominantly localized in the PM before activation [34] , while the majority of CRT1 is in endomembranes [13] , an interesting question is where these immune proteins interact. Analyses of endoglycosidase H sensitivity [35] have suggested that FLS2, whether expressed in N. benthamiana or Arabidopsis , is present in both the endoplasmic reticulum and PM [36] , [37] . Moreover, a portion of FLS2 was found in endomembranes [36] , suggesting the CRT1–FLS2 interaction may occur in this compartment. Supporting this possibility, the animal PRRs TLR9 and TLR4, key factors in modulating innate and adaptive immunity, require localization to endosomes for their functions [38] , [39] . Interestingly, TLR4 mediates defence signalling by interacting with MyD88 and TRIF in the PM and endosomes, respectively; the MyD88- and TRIF-dependent pathways function synergistically when both are activated [40] . Therefore, it is plausible that CRT1 functions together with FLS2 in endomembranes, whereas a PM-associated population of FLS2 acts through another pathway, perhaps in a synergistic manner. Nuclear translocation of R proteins and several downstream immune components, including NPR1 and EDS1, has a critical role in plant immunity [41] . CRT1’s translocation to the nucleus upon activation of R/PRR proteins strongly suggests a nuclear role(s) for CRT1 in disease resistance. One possible function might be in DNA R/R. Although the importance of DNA R/R in disease has only recently begun to be appreciated in plants and humans [42] , [43] , emerging evidence suggests that R/R is involved in pathogen-induced transcriptional reprogramming. For instance, SNI1 (Suppressor of NPR1, Inducible) was proposed to mediate defence gene expression via histone modification [44] . Interestingly, several ssn mutants encode mutated versions of well-established DNA R/R proteins, such as RAD51D (SSN1), SWI/SNF (SSN2) and BRCA2A (SSN3) [30] , [45] , [46] . Mutations in any of the three SSN genes results in altered induction of pathogen-responsive genes and increased susceptibility/sensitivity to pathogens and DNA-damaging agents. The combined findings that (i) CRT1 exhibits endonuclease activity, (ii) nuclear CRT1 levels increase following R/PRR activation and (iii) crt1-2 crh1-1 displays enhanced tolerance to mitomycin C, suggest that the CRT1 family also functions in modulating DNA R/R, perhaps as a negative regulator, following immune receptor activation. Please note that although tolerance to DNA-damaging agents is reduced in the ssn mutants and enhanced in our dKO, both sets of mutants are compromised for disease resistance. Two independent screens for mutants that are suppressed for gene silencing recently identified CRT1 and its homologue CRH6. Mutations in either of these genes restored the previously silenced expression of a GFP transgene [19] , [20] . These findings suggest that CRT1 directly or indirectly modulates RNA silencing. RNA silencing is a critical component of plant immune responses against viral and bacterial pathogens [47] . Many viruses, including TCV, encode proteins that disrupt this defense [48] . In plants, the small RNAs involved in RNA silencing have critical roles in reprogramming host gene expression following infection with various pathogens [49] , [50] , [51] , [52] . Thus, CRT1-mediated RNA silencing may be responsible for at least some of these host responses although most of the defence genes tested were not affected by CRT1/CRH1 ( Supplementary Fig. S2 ). It remained to be determined whether functionally redundant CRH2 may have obscured PTI-associated transcriptome changes in dKO. Although eukaryotic MORC proteins are associated with DNA/chromatin modification [16] , there is no prior evidence suggesting MORC protein involvement in immunity. However, the association of prokaryotic MORCs with restriction–modification systems, an ancient defence system that discriminates nonself from self DNA, is consistent with this possibility [16] . Here we show for the first time that a eukaryotic MORC, CRT1, is a critical factor in multiple levels of plant immunity. Furthermore CRT1’s biochemical activities and differential localization to the nucleus after pathogen challenge suggest that it likely functions in chromatin/DNA modification, which may affect transcriptional reprogramming. Given that transposons and other silenced genes are derepressed in the crt1 and crh6 mutants [19] , [20] , and that infection can induce genome instability [53] , which may result from derepression of transposons, we propose that enhanced mobilization of CRT1 to the nucleus after pathogen infection may help regulate transcriptional reprogramming and also maintain genome stability, in part by suppressing the derepression of transposons and/or other silenced genes. DNA constructs Plant overexpression constructs for Myc-CRT1 (ref. 12 ) and Myc-GFP [54] were described previously. A DNA fragment encoding the triple Flag epitope with Sal I and Xho I sites was ligated into pER8, creating pER8-Flag; an Asc I site was added to the 5′ end of the Flag tag. FLS2 with Asc I sites at each end was amplified from Arabidopsis cDNA with the oligonucleotides: 5′-GGCGCGCCATGAAGTTACTCTCAAAGACCTTT-3′ and 5′-GGCGCGCCAACTTCTCGATCCTCGTTACGATC-3′. Amplified FLS2 fragment was ligated into pER-Flag, creating pER-FLS2-Flag. To generate Myc-gCRT1 , the promoter of CRT1 with PacI and AscI sites at each end was amplified using BAC F23E13 and the oligonucleotides: 5′-TTAATTAAACTTCTTTAGTCGTTGGTTTCATT-3′ and 5′-GGCGCGCCTACCGACGGCGACAAAACGAATTC-3′. pER- Myc-CRT1 (ref. 12 ) was digested with Asc I and Xho I, to provide a fragment carrying the 6 × Myc tag and the first 155 bp of CRT1 ; note that the genomic sequence corresponding to this fragment does not have an intron, and Xho I is a unique site present in CRT1 . The 3′ portion of CRT1 was isolated by digesting BAC F23E13 DNA with Xho I and Xba I; the Xba 1 site is located 80 bp 5′ to the initiation codon for the neighbouring gene, CRH1 . These three fragments were sequentially cloned into pPZP-RCS1 carrying a hygromycin resistance marker ( hpt ) using Pac I, Asc I, Xho I and Xba I sites [55] , to create pPZP- Myc-gCRT1 . The putative CC domain (511–635 a.a.) of CRT1 amplified using the oligonucleotides: 5′-GAATTCGTCTGATAGAATCAGTCATGGTGGTC-3′ and 5′-CTCGAGCTAAACTTGTTGCATCTCCTTCTT-3′ was ligated into pET28b, creating pET28b-CRT1-CC. Co-IP and IB analyses and generation of transgenic plants Agrobacterium -mediated transient expression in N. benthamiana and Agrobacterium -mediated transformation of Arabidopsis were performed as described [12] . Co-IP and IB were performed as described [12] . Equal loading of proteins was checked by staining the polyvinylidene difluoride membrane (Millipore) with Coomassie blue to visualize the large subunit of RuBPCase or by analysing IB with αPEPC (Rockland). Pathogen infection assays To examine flg22-induced resistance, the leaves of 4-week-old Arabidopsis plants were infiltrated with water or 0.2 μM flg22 peptide (Genscript). After 24 h, the same leaves were infiltrated with 10 5 c.f.u. ml −1 of Pst DC3000. Bacterial growth was determined 3 d.p.i. as previously described [12] . TCV inoculation on 4-week-old plants was performed as described [12] . For P. infestans inoculation, isolate US050007, corresponding to the US-11 genotype, was grown on rye B agar at 15 o C and the oomycete sporangia were harvested by washing the plates with sterilized water. The suspension was adjusted to 10 5 sporangia per ml and incubated for 3 h at 4 °C for zoospore release. Four-week-old Arabidopsis plants were sprayed with the sporangia suspension until every leaf appeared evenly wet. Plants were grown at 16 °C with a 16 h-day cycle on trays with a cover to maintain high humidity. RNA extraction and quantitative real-time RT–PCR RNA extraction and quantitative real-time RT–PCR was performed as described [13] . The primers for CRA genes [13] and PTI-associated genes [25] were described previously. Each of three biological replicates was analysed in duplicate. Root extension and ROS generation assay The root extension assay in the presence of flg22 or water was performed as previously described [23] . The ROS generation assay in the presence of flg22 or water was performed as previously described [56] . Data quantitation for SA measurements and stainings SA was extracted and quantified from inoculated leaves as previously described [57] . Trypan blue staining was performed as described previously [12] . Photographs were taken using an Olympus SZX-12 Stereo Microscope. Aniline blue staining was carried out as described previously [58] . Photographs were taken using a Leica DM5500 Epifluorescence Microscope. Cell death, callose deposition and gel images were quantified using the ImageJ (NIH). Expression and purification of recombinant CRT1 Recombinant CRT1 and CRT1-CC (511–653 a.a.) proteins were expressed in Escherichia coli using pET28b-CRT1 or pET28b-CRT1-CC and purified as previously described, except the following modifications [12] . E. coli strain BL21 cells carrying the respective plasmids were grown at 37 °C to OD 600 =0.7. Expression of CRT1 was induced by adding 0.1 mM isopropyl-β- D -thiogalactoside for 20 h at 18 °C. The collected cells were resuspended in lysis buffer, buffer A (25 mM HEPES/7.5, 0.5 M NaCl, 2 mM dithiothreitol (DTT), 10% glycerol) containing 10 mM imidazole and phenylmethyl sulphonyl fluoride. After sonication and centrifugation (1 h, 50,000 g , 4 °C), the soluble 6 × His-tagged CRT1 protein was purified by affinity chromatography using Ni-NTA agarose resin (Novagen); following washing the CRT1-bound resin with buffer A containing 20 mM imidazole, CRT1 was eluted in buffer A containing 300 mM imidazole. The eluted CRT1 was subjected to gel filtration chromatography on a HiLoad 16/60 Superdex 200 column (GE Healthcare) equilibrated in buffer B (50 mM Tris–HCl/7.5, 300 mM NaCl, 2 mM DTT, 10% glycerol). The fraction containing highest amount of purified CRT1 was further purified using anion exchange chromatography on a SOURCE 15Q 4.6/100 PE column (GE Healthcare) equilibrated in buffer C (25 mM Tris–HCl/8.0, 2 mM DTT, 10% glycerol). After washing with buffer C containing 125 mM NaCl, CRT1 was eluted with buffer C containing 500 mM NaCl. In vitro endonuclease assay Ten microlitre of reaction mixture contained 200 ng arbitrary supercoiled plasmid DNA, pER8-HA [12] , in 50 mM Tris-HCl/8.0, 1 mM DTT and 10 mM metal salt (MgCl 2 , MnCl 2 or ZnCl 2 ). Reactions were incubated at 37 °C for varying lengths of time, terminated by addition of an equal volume of 2 × stop buffer (2% SDS, 100 mM EDTA, 20% glycerol and 0.2% bromophenol blue), and then electrophoresed on a 1.2% agarose gel at 4 V cm −1 with 1 × TAE running buffer. Plant material preparation and TEM analysis Plants were grown in soil at 22 °C, 60% relative humidity (RH), and a 16 h light period. Intercellular spaces of leaves from 6-week-old crt1-2 crh1-1 and Myc-gCRT1 plants were flooded with 5 μM flg22 or 10 mM MgCl 2 (mock) via syringe infiltration. Collected leaves were cut into samples of about 5 × 5 mm. Immunocytochemistry was performed as previously described [59] with the following modifications: Tannic acid (0.5% w/v) was added to the fixative. Sections were incubated for 2 h with αMyc antibody (Roche) diluted 1:400 (v/v) in 0.1 M PBS with 0.5% (w/v) BSA, followed by treatment with 5 nm gold-labelled αMouse IgG (Sigma) diluted 1:50 (v/v) in 0.1 M PBS with 0.5% (w/v) BSA for 1.5 h. Post-stain samples were examined in a LEO EM 912 (Zeiss) TEM at 120 kV. Digital micrographs were taken with an integrated charge-coupled device camera (Proscan). Figures were composed using Corel Photo Paint 10. Subcellular fractionation and fluorescence spectrometry Enrichment of plant nuclei was performed as previously described [60] . For fluorescence spectrometry, the protein solution of purified CRT1 was adjusted to a concentration of 10 μg ml −1 . Following excitation at 280 nm, the emission spectra of CRT1 in the absence or presence of nucleic acid (100 ng λ-phage DNA, a plasmid carrying TCV DNA, TCV in vitro transcript or yeast RNA) were recorded from 300 to 400 nm at 20 °C with the band width set to 5 nm. Spectra were accumulated and averaged three times at an acquisition speed of 0.5 nm, and subsequently buffer-corrected. Spectra of the native protein were recorded in buffer B (see expression and purification of recombinant CRT1). For denaturation, the protein solution was exposed to repeated freeze–thaw cycles. How to cite this article: Kang, H-G. et al. CRT1 is a nuclear-translocated MORC endonuclease that participates in multiple levels of plant immunity. Nat. Commun. 3:1297 doi: 10.1038/ncomms2279 (2012).